RETRACTED ARTICLE:Endocrine disruptors induce perturbations in endoplasmic reticulum and mitochondria of human pluripotent stem cell derivatives Persistent exposure to man-made endocrine disrupting chemicals during fetal endocrine development may lead to disruption of metabolic homeostasis contributing to childhood obesity. Limited cellular platforms exist to test endocrine disrupting chemical-induced developmental abnormalities in human endocrine tissues. Here we use an human-induced pluripotent stem cell-based platform to demonstrate adverse impacts of obesogenic endocrine disrupting chemicals in the developing endocrine system. We delineate the effects upon physiological low-dose exposure to ubiquitous endocrine disrupting chemicals including, perfluoro-octanoic acid, tributyltin, and butylhydroxytoluene, in endocrine-active human-induced pluripotent stem cell-derived foregut epithelial cells and hypothalamic neurons. Endocrine disrupting chemicals induce endoplasmic reticulum stress, perturb NF-κB, and p53 signaling, and diminish mitochondrial respiratory gene expression, spare respiratory capacity, and ATP levels. As a result, normal production and secretion of appetite control hormones, PYY, α-MSH, and CART, are hampered. Blocking NF-κB rescues endocrine disrupting chemical-induced aberrant mitochondrial phenotypes and endocrine dysregulation, but not ER-stress and p53-phosphorylation changes. Of the thousands of chemicals to which Americans are exposed, only about 2% of the chemicals have undergone a safety review by government scientists. Only recently, a bipartisan reform passed by the US congress overhauled the effectively weak 1976 Toxic Substances Control Act (TSCA) that governs the introduction and use of industrial chemicals. A subset of these pervasive environmental pollutants, known as endocrine disrupting chemicals (EDCs), target hormonal control of hunger and satiety [1] , [2] , disrupt normal tissue development, and interfere with the body’s homeostatic controls [3] , [4] , [5] . Repeated exposures of these “obesogenic” EDCs during critical windows of stem cell development in utero can alter some genetically pre-disposed individuals’ normal metabolic control, and set them up for long-term obesity. Transgenerational exposure of EDCs from mother to the offspring also brings about adverse epigenetic imprinting effects during critical embryonic stem cell development [6] . Strong evidence suggests that such exposure of EDCs during early development impart detrimental life-long effects on endocrine physiology and normal metabolic homeostatic controls [7] , [8] . EDCs alter basal metabolic rate by shifting energy balance and promoting calorie storage [9] , thereby contributing to obesogenic phenotypes. Further, increased body mass index and obesity may be inherited across generations due to maternal obesity during gestation [10] . Barring a few instances of genetic causes of obesity, a slew of biological and behavioral factors affects energy balance [11] . Genome-wide association studies (GWAS) have identified multiple obesity-associated loci [12] , some of which have been validated in the animal models. Assuming that the human gene pool has not changed as expeditiously as the upsurge in childhood obesity, the chemical environment interacting with an individual’s genetic background, is a significant driver modifying the risk and severity of obesity. Better elucidations of disruptions after exposure of EDCs and other industrial chemicals are warranted in faithful human cell models, without solely relying on tumor cell lines or animal models. To fill this void, we employed human-induced pluripotent stem cells (hiPSCs) and elucidated the adverse effects of chronic low-dose EDC exposures on developing gut endocrine and hypothalamic neuroendocrine cells. Endocrine control of feeding behavior involves the communication between the hypothalamic arcuate nucleus and the gastrointestinal (GI) tract. The hypothalamic (HT) neuropeptidergic neurons receive endocrine signals from parts of gut including gastrin and ghrelin from stomach, peptide YY from midgut and intestine [13] among others, and bring about orexigenic or anorexigenic responses. Hence, perturbations during development due to environmental factors such as EDCs may have a role in dysfunction of the gut–brain interactions thereby bringing about feeding disorders and obesity. Although couple of reports described generation of a population of hypothalamic neurons from PSCs, albeit at low efficiencies [14] , [15] , we utilized an efficient serum-free and chemically defined method for differentiation of iPSC-derived hypothalamic neuronal cultures (>85% neurons) without complex selection procedures. Previous studies have also described derivation of three-dimensional (3D) stomach and intestinal organoids from pluripotent stem cells [16] , [17] . In this manuscript, we show ability to culture gut organoids as adherent monolayers of gut epithelium, thus making them amenable to toxicology and endocrine function assays. Here, we apply these hiPSC-derived endocrine culture systems concomitantly as a relevant human developmental models for screening endocrine perturbations. We describe the effects of three different EDCs—perfluoro-octanoic acid (PFOA), tributyltin (TBT), and butylhydroxytoluene (BHT)—at physiologically relevant concentrations in developing human endocrine tissues. PFOA is a fluoropolymer surfactant known to persist indefinitely in the environment. About 98% of the US population has detectable levels of PFOA in their blood [18] , likely exposed through water, industrial waste, stain resistant carpets, house dust, water, and cookware coating [19] . Epidemiological studies on PFOA exposure are correlated with higher cholesterol levels, thyroid disease, ulcerative colitis, and reproductive insufficiencies [20] . A few studies show increased incidence of elevated total cholesterol levels (0.25–17,557 ng/mL serum level) [21] , increased hazards of cancer [22] (0.25–22,412 ng/mL) [23] . On the basis of these and other animal studies [24] , [25] , [26] , we studied the consequences of 2.5 µM (1035.175 ng/mL) PFOA as a relevant physiological level low dose. TBT, an organotin, is used as an anti-fouling agent used in paints [27] is also largely present in house dust and water [28] , and its bioaccumulation in seafood has posed the most exposure risk to humans. The current estimated daily intake for TBT is 0.25–2.5 µg/kg body weight [29] . Thus, 10 nM TBT was used here based on existing literature on thyroid hormone response [30] , [31] . BHT, a common food additive and an ingredient in personal care cosmetics, pesticides, plastic, and rubber [32] , is also utilized as an antioxidant in commonly consumed breakfast cereal brands [33] . The mean intake is between 0.7 and 0.99 mg/kg bodyweight (240% of admissible daily intake levels) [34] . However, with no relevant in vitro toxicity data available for BHT, a low-dose of 10 nM BHT was utilized. There is a paucity of data on human developmental abnormalities and underlying mechanisms of cellular dysfunction in appetite and satiety pathways upon early exposure to EDCs, largely due to the implausibility of accessing developing human fetal tissue [11] , [35] . In this study, we demonstrate that EDCs induce endoplasmic reticulum (ER) and metabolic stress in relevant human endocrine tissues perturbation of NF-κB and p53 signaling, reduced transcription of both nuclear-encoded and mitochondrial-encoded respiratory genes, defective mitochondrial respiration, decreased ATP levels, and subsequent peptide hormone dysregulation. The human stem cell platform described here provides an advantage for screening the effect of early human exposure to EDCs. Reprogramming of blood mononuclear cells to pluripotency Non-integrating reprogramming of peripheral blood mononuclear cells (PBMCs) to iPSCs was performed using the episomal (OriP/EBNA1) plasmid-based method similar to published protocols in our lab [36] , [37] . This included nuclear transfection of seven transient and episomally expressed reprogramming factors OCT3/4 , SOX2 , KLF4 , LIN28 , non-transforming L-MYC , SV40 large T antigen ( SV40LT ), and shRNA against TP53 (Supplementary Fig. 1a ). This protocol resulted in successful generation of blood-derived non-integrating iPSC clones that could be mechanically isolated and expanded after 27–32 days (Supplementary Fig. 1a ). Representative images from independent iPSC lines used in this study (80iCTR Tn2 and 201iCTR NTn4) exhibited typical features of hPSCs such as tight colonies with high nucleus to cytoplasm ratio (Supplementary Fig. 1b ). They also exhibit robust alkaline phosphatase activity, and strong expression of nuclear (OCT3/4, NANOG, SOX2) and surface (SSEA-4, TRA-1-81, TRA-1-60) pluripotency proteins (Supplementary Fig. 1b ). The PBMC-iPSCs also passed the PluriTest assay with high pluripotency and low novelty scores (Supplementary Fig. 1c ) and maintained normal cytogenetic status (Supplementary Fig. 1d ). OriP/EBNA1 vectors replicate just once per cell cycle, and in the absence of drug selection, the episomes are lost at the rate of 5% per generation and cells are rendered plasmid-free [38] (Supplementary Fig. 1e , f). Thus, this episomal reprogramming method employed here does not interfere with any cellular molecular mechanisms including the expression of TP53 gene (Supplementary Fig. 1g ). iPSCs differentiate into endocrine-active foregut epithelium On the basis of the 3D gastric organoid differentiation previously published [16] , we adapted and modified this method to generate two dimensional monolayers of gastric epithelium with endocrine abilities. In a stepwise method, human iPSC cultures were successfully specified into foregut epithelium containing endocrine cell types by first patterning definitive endoderm with activin A and Wnt3A ligands, followed by simultaneous activation of WNT (CHIR), FGF (FGF4), and retinoic acid (RA) signaling while repressing BMP signaling. Finally, foregut epithelium composed of endocrine cells was obtained by stimulating with high concentrations of epidermal growth factor (EGF) (Fig. 1a ). After definitive endoderm induction, at 6 days’ post-iPSC, gut-tube organoid structures emerged from the endoderm monolayer. Upon re-plating the gut-tube organoids, an adherent epithelial-shaped cell layer consistently emerges between 7 and 20 days post-iPSCs (Fig. 1b ). Monitoring expression of relevant foregut-specific genes confirmed the characterization of iPSC-derived foregut epithelium (iFGE) at day 20. Significant gene expression of SOX2 (foregut progenitor), PDX1 (antral foregut), GKN1 ( gastrokine 1; gastric mucosa), PGA5 (digestive enzyme), TAS1R3 (taste receptor in the foregut), and TFF2 (trefoil factor 2; stable secretory protein of gastric mucosa) in the foregut were observed in the adherent iFGEs (Fig. 1c ). It is important to note that the iFGEs did not exhibit expression of hindgut-specific transcription factor, CDX2 (Fig. 1c ) and were consistently positive for epithelial cell surface-specific proteins, CDH1 (E-cadherin) and CTNNB (β-catenin) (Fig. 1d ). Endoderm and foregut progenitor-specific transcriptional factors, Sox17 and Sox2, respectively, confirm the foregut identity of the iFGEs (Fig. 1d ). Importantly, neuroendocrine markers known to be present in endocrine-active foregut such as synaptophysin (SYP), somatostatin, and serotonin were expressed by the iFGE at day 20 (Fig. 1e ). Notably, the iFGEs were also immunopositive for stomach-specific hormone-expressing enteroendocrine cells like gastrin (G cells), ghrelin (parietal cells), and a few peptide YY (mucosal) L cells (Fig. 1f ). Fig. 1 Human iPSCs differentiate into foregut epithelium (iFGE) by modulation of WNT, FGF, BMP, and RA. a iFGE differentiation protocol. b Bright field images of day 6 and day 20 old iFGE. c RT-qPCR of foregut genes shown to be significantly increased (** p < 0.01) in day 20 iFGE compared with day 0. ND not detectable. Two-way ANOVA was employed to determine differences within day 0 and day 20 iFGEs. d Foregut epithelial markers, E-cadherin (CDH1), β-catenin (CTNNB), and endoderm and foregut progenitor markers, Sox2 and Sox17. e Expression of neuroendocrine markers such as synaptophysin (SYP), somatostatin and serotonin. f ( Top to bottom ) Gastric endocrine-positive cells such as ghrelin, peptide YY, and gastrin. All markers from d , e , and f are co-labeled with an epithelial marker such as E-cadherin ( red ) or β-catenin ( green ). Images and data shown are representative of average results from the two iPSC lines differentiated n = 5 times in independent experiments. Scale bars represent 50 µm. Error bars denote s.e.m Full size image Neuropeptidergic hypothalamic neurons from iPSC The neuropeptidergic hypothalamic neurons (iHTNs) were generated after directed neuroepithelia specification upon dual SMAD inhibition (SMADi) of iPSCs [39] . Subsequently, early WNT inhibition and SHH activation specified forebrain cell types of ventral diencephalon identity where the hypothalamus and the arcuate nucleus (ARC) resides [15] , [40] (Fig. 2a ). Synchronizing the forebrain progenitors and terminal maturation of the differentiating neurons yielded increased expression of hypothalamic and neuropeptidergic genes such as AgRP ( Agouti-related Peptide ; an orexigenic neuropeptide), MC4R ( Melanocortin 4 receptor ; regulation of feeding and metabolism), Nkx2.1 (ventral diencephalon marker), NPY ( Neuropeptide Y ; orexigenic neuropeptide co-expressed with AgRP ), and PCSK2 ( Proprotein Convertase Subtilisin/Kexin Type 2; neuroendocrine gene) (Fig. 2b ). The secretion of hypothalamic neuropeptides, NPY, and α-melanocyte-stimulating hormone (α-MSH), revealed significantly higher levels of secreted neuropeptides in day 40 iHTNs (Fig. 2c, d ). Presence of several neuroendocrine and hypothalamic ARC-specific proteins like OTP (homeobox protein orthopedia; Fig. 2e ), α-MSH (Fig. 2f ), NPY (Fig. 2g ), SST (somatostatin; Fig. 2h ), GABA (Fig. 2i ), CPE (carboxypeptidase E; Fig. 2j ), CART (Cocaine-regulated and amphetamine-regulated transcript; Fig. 2k ), NP-II (neurophysin II/arginine vasopressin; Fig. 2l ), 5-HT (serotonin; Fig. 2m ), and TH (tyrosine hydroxylase; Fig. 2n ) were observed. Electrophysiological measurements using multi-electrode arrays (MEAs) shows regular trains of spontaneous action potentials and repetitive firing in day 40 iHTNs, thus confirming a bona fide neuronal identity and electrical maturity of iHTNs (Fig. 2o ). Fig. 2 Functional neuropeptidergic hypothalamic neurons (iHTNs) can be derived from hiPSC. a iHTN differentiation protocol. b RT-qPCR of hypothalamic and arcuate nucleus-specific genes showing significantly increased expression of the genes at day 40 of differentiation compared with day 0 (* p < 0.05, ** p < 0.01). ND not detectable; two-way ANOVA was employed to determine differences within day 0 and day 40 iHTNs. c Measurement of hypothalamus-specific neuropeptide Y ( NPY ) measured from cell supernatants using ELISA ( p < 0.001 determined using paired t -test). d Measurement of hypothalamus-specific α-melanocyte-stimulating hormone (α-MSH) measured from cell supernatants using ELISA (*** p < 0.001 determined using paired t -test). e – n Immunopositivity for hypothalamic progenitors and neuropeptidergic markers. o MEA readings of neurons from day 0 as well as day 40 from the same electrode over time showing increased neuronal firing in day 40 neurons. Images and data shown are representative of average results from the two iPSC lines differentiated n = 5 times in independent experiments. Scale bars represent 50 µm. Error bars denote s.e.m Full size image EDCs induce ER stress but not cell death After successful differentiation of iPSC-endocrine cell cultures, we perturbed these tissues with EDCs at low-dose over a 12-day treatment paradigm (Fig. 3a, b ). The concentrations for EDC treatments were selected based on; (i) between one log and semi-log below the dose at which ≤10% loss in cell viability was observed compared with untreated controls (Supplementary Fig. 2a–f), and (ii) the human tolerable daily intake (TDI) ranges of each EDC based on ToxCast database and literature. Accordingly, we performed individual treatments of perfluoro-octanoic acid (PFOA; 2.5 μM), tributyltin (TBT; 10 nM), and butylhydroxytoluene (BHT; 10 nM), along with combination treatment paradigm that is like concomitant environmental exposure to multiple EDCs (Supplementary Fig. 2a–f ). Fig. 3 Chronic low-dose EDC treatment induces ER stress in iFGEs and iHTNs without affecting cell viability. a A schematic representation of EDC treatments and analysis performed on iFGEs and iHTNs. b A schematic showing the kinetics of EDC treatments performed on iFGEs and iHTNs. c , d Representative immunoblots showing levels of bona fide ER-stress pathway proteins, IRE1, BiP, and Ero1, in c iFGE and d iHTNs. Quantified histograms using ImageJ-based densitometry of bands for each of the respective protein immunoblots normalized to Cox IV as loading control are shown below and represented as fold-change compared with vehicle-treated control. IRE1 protein increases, whereas BiP and Ero1 levels decrease in response to EDC exposure, * p < 0.05, ** p < 0.01, *** p < 0.001. e , f MTT assay shows no significant differences in cell viability upon EDC exposure in both e iFGEs and f iHTNs. All statistical analyses were performed using one-way ANOVA. Data shown are representative of average results from the two iPSC lines differentiated n = 3 times in independent experiments. Error bars denote s.e.m Full size image Treatment of iFGEs and iHTNs with EDCs, engendered disturbances in levels of ER stress sensor proteins. EDCs increased ER transmembrane stress sensor protein, inositol-requiring enzyme 1 (IRE1), known to activate the unfolded protein response (UPR), between 1.5-fold and 2-fold (Fig. 3c, d ). The molecular chaperone, binding immunoglobulin protein (BiP)/GRP78, was decreased between 0.4-fold and 0.5-fold in expression upon EDC treatment. BiP binds to misfolded proteins to prevent them from forming aggregates and assists in proper refolding (Fig. 3c, d ). Secretory and transmembrane proteins translocated into ER that are modified by disulfide bond formation, amino-linked glycosylation and folding, require BiP to fold properly. When BiP levels decrease, native protein folding confirmation is severely perturbed. Another ER membrane-associated N -glycoprotein, Ero1 (ER oxidoreductin1), responsible for post-translational intra-molecular and inter-molecular disulfide bonds and protein folding, was significantly attenuated upon EDC treatment by about 0.4-fold to 0.6-fold (Fig. 3c ). Many secreted proteins undergo oxidative protein folding process mediated by Ero1 to reach their native conformation. Altogether, this points towards an activation of an early ER stress pathway by low-dose EDC treatment in developing endocrine cells. Importantly, the resulting changes in ER stress sensor proteins were neither a consequence of EDC-induced cytotoxicity or loss in cell viability (Fig. 3e, f ), nor any significant negative impacts of EDC treatments on differentiation capacity of the endocrine cell cultures (Supplementary Fig. 3 ). The latter was assessed by performing histological cell counts of epithelial marker, E-cadherin (Supplementary Fig. 3a ), in the iFGE cultures, and OTP and Tuj1 (β III -tubulin) (Supplementary Fig. 3b ), AgRP (Supplementary Fig. 3c ), NPY (Supplementary Fig. 3d) , α-MSH (Supplementary Fig. 3e ), and POMC (Supplementary Fig. 3f ), in the iHTNs. Chronic low-dose EDC treatment perturbs NF-κB signaling Evidence supports perturbation of NF-κB signaling upon activation of ER stress and the UPR pathways [41] , [42] , [43] , [44] , [45] , [46] . Upon treatment with EDCs in developing iPSC-derived endocrine tissues, a significant increase in phosphorylated NF-κB p65 (RelA) immunopositive cell numbers was observed in iFGE cells from 1.35-fold to 1.5-fold and 1.2 to 1.3-fold in iHTNs (Fig. 4a ) ( p < 0.001; one-way ANOVA). Immunoblotting of these cultures confirmed that NF-κB p65 phosphorylation levels were shown to be significantly elevated in EDC-treated iFGEs (Fig. 4b ) ( p < 0.001; one-way ANOVA) and iHTNs (Fig. 4c ) ( p < 0.01; one-way ANOVA) (Supplementary Fig. 4 ). Phosphorylation of NF-κB p65 is required for dimerization with p50 and translocation to the nucleus [47] . As p65 (RelA) activation was observed with EDC treatment, activation of the canonical NF-κB pathway was assessed by determining the ratio of the active p50 form to the inactive p105 (NF-κB1) subunit. The dimerization of p50 with the phosphorylated p65 subunit and subsequent proteasomal degradation of IκBα leads to the typical nuclear translocation of p65–p50 dimers [48] , [49] , thus resulting in the transcriptional regulation of κB-dependent genes. Upon individual and combination EDC treatments, p50 levels were higher in relation to its precursor p105, which shows activation of the canonical pathway in EDC-treated iPSC-endocrine cultures. Interestingly, both iFGEs and iHTNs showed EDC-mediated increase in p50/p105, (Fig. 4b, c ) ( p < 0.001; one-way ANOVA). In a similar approach to determine the involvement/activation of the non-canonical NF-κB pathway, we measured the ratio of protein expression of p100 to p52. Briefly, the non-canonical NF-κB pathway involves the dimerization of RelB and p52, and hence a measure of the amount of p52 indicates the possible activation of this pathway. We observed significant increases in the ratio of p52/p100 with the treatment of EDCs in both iFGE (1.4-fold to 2-fold; p < 0.001; one-way ANOV) (Fig. 4b ) and iHTN (1.5-fold to 2.5-fold; p < 0.001; one-way ANOVA) (Fig. 4c; Supplementary Fig. 5 ). Thus, to the best of our knowledge, this is the first report demonstrating that EDCs significantly perturb the NF-κB pathway in endocrine-active human cells. Fig. 4 EDC treatment causes disturbances in NF-κB p65 canonical and non-canonical pathways. a Top panel : representative immunocytochemistry ( ICC ) showing increases in phosphorylated p65 ( red ) in iFGEs co-stained with ghrelin ( green ). Bottom panel : representative ICC showing increases in phosphorylated p65 ( red ) in iHTNs co-stained with synaptophysin ( green ) (*** p < 0.001). Immunopositive cells were scored and quantified in histograms for both iFGEs and iHTNs, which is represented by fold-change in phosphorylated NF-κB p65 immunopositive cells in each of the EDC treatments compared with the vehicle control-treated iFGEs (*** p < 0.001) and iHTNs (*** p < 0.001). Representative immunoblots for protein levels in whole-cell lysate showing increases in phosphorylated p65, total p50, and total p52 levels in b iFGE, *** p < 0.001 and c iHTNs *** p < 0.001. Quantified histograms using ImageJ-based densitometry of bands for each of the respective immunoblots are shown below and represented as fold-change compared with vehicle-treated control. Ratio of phosphorylated NF-κB p65 over total p65, p50/105 (canonical), and p52/p100 (non-canonical) were calculated. All statistical analyses were performed using one-way ANOVA. Images and data shown here are representative of average results from the two iPSC lines differentiated n = 3 times in independent experiments. Scale bars represent 50 µm. Error bars denote s.e.m Full size image EDCs disrupts p53 signaling, mitochondria, ATP and hormone levels ER stress and disturbances in both NF-κB and p53 signaling impair mitochondrial function, both by directly and indirectly regulating transcription of relevant nuclear-encoded and mitochondrially encoded respiratory genes [50] . Thus, we determined whether chronic EDC exposure adversely impacts p53 signaling and mitochondrial function in human endocrine tissues. It was found that phosphorylated p53 (Pp53 at Ser15) levels were significantly decreased in EDC-treated samples when compared with the untreated controls (p < 0.001; one-way ANOVA) in iHTNs as well as in iFGEs ( p < 0.001; one-way ANOVA) (Fig. 5a ). Fig. 5 EDCs induce metabolic stress and disrupt endocrine regulation. a Immunoblots showing decreases in phosphorylated p53 (Ser15) in both iFGEs and iHTNs (*** p < 0.001) upon EDC exposure. b Seahorse mitochondrial respirometry measurements with histograms representing changes in spare respiratory capacity in iFGEs and iHTNs, * p < 0.05; ** p < 0.01. c Relative normalized expression of nuclear ( SCO2, POLRMT, TFAM ) and mitochondrial-encoded ( CYB5A ) genes involved in mitochondrial respiration in iHTNs as measured by RT-qPCR. d Measurement of ATP levels (ATP/ADP ratio) showing decreases with EDC treatments. e Immunoblots showing decreases in PYY levels in EDCs-treated iFGEs. f ELISA of α-MSH showing decreases in secretion with EDC treatment of iHTNs. * p < 0.05, ** p < 0.01, *** p < 0.001, n = 3. ND not detectable. All statistical analysis was performed using one-way ANOVA. Data shown here are representative of average results from the two iPSC lines differentiated n = 3 times in independent experiments. Error bars denote s.e.m Full size image Next, the effects of EDCs on mitochondrial respiration were determined by performing a mitochondrial stress test using the extracellular flux technology. BHT ( p < 0.05; one-way ANOVA) addition and combination treatment of PFOA, TBT, and BHT ( p < 0.01; one-way ANOVA) decreased maximal respiration and spare respiratory capacity by 40–50% in iFGEs (Fig. 5b ). Similarly, combination, TBT, BHT treatments in iHTNs exhibited a 40–50% decrease in maximal respiration and spare respiratory capacity (Fig. 5b ). Changes or a loss in mitochondrial mass was ruled out as result of EDC exposure, as the COX IV (inner mitochondrial membrane enzyme) levels between all treatments did not vary (Supplementary Fig. 6 ). Further, the transcriptional regulation mechanism behind this mitochondrial impairment was deduced by examining gene expression levels of critical nuclear-encoded mitochondrial respiratory genes such as SCO2 (Cytochrome C oxidase 2), POLRMT (Mitochondrial RNA polymerase), TFAM (transcription factor A, mitochondrial), and mitochondrially encoded CYB5A (Cytochrome B5). EDC treatments significantly and negatively influenced expression of critical respiratory genes in both iFGEs (Supplementary Fig. 7 ) and iHTNs (Fig. 5c ). SCO2 , POLRMT , TFAM , and CYB5A gene expression upon individual EDC treatment was downregulated, with combination treatment eliciting the most significant decrease in these transcripts. 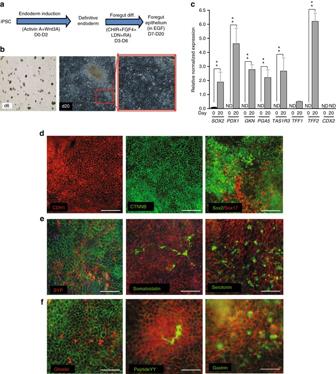Fig. 1 Human iPSCs differentiate into foregut epithelium (iFGE) by modulation of WNT, FGF, BMP, and RA.aiFGE differentiation protocol.bBright field images of day 6 and day 20 old iFGE.cRT-qPCR of foregut genes shown to be significantly increased (**p< 0.01) in day 20 iFGE compared with day 0.NDnot detectable. Two-way ANOVA was employed to determine differences within day 0 and day 20 iFGEs.dForegut epithelial markers, E-cadherin (CDH1), β-catenin (CTNNB), and endoderm and foregut progenitor markers, Sox2 and Sox17.eExpression of neuroendocrine markers such as synaptophysin (SYP), somatostatin and serotonin.f(Toptobottom) Gastric endocrine-positive cells such as ghrelin, peptide YY, and gastrin. All markers fromd,e, andfare co-labeled with an epithelial marker such as E-cadherin (red) or β-catenin (green). Images and data shown are representative of average results from the two iPSC lines differentiatedn= 5 times in independent experiments.Scale barsrepresent 50 µm.Error barsdenote s.e.m Bioinformatics analysis identifying putative-binding motifs near the transcription start sites of SCO2 , POLRMT , TFAM , and CYB5A for the RelA (p65) and TP53 (p53) as transcription factors suggests that NF-κB could directly regulate the transcription of these mitochondrial respiratory genes (Table 1 ; Supplementary Tables 1 and 2 ; Supplementary Fig. 8 ). Although less in number, p53 also has transcription factor binding sites for these genes, thus potentially regulating their transcription. Notably, both p53 and NF-kB p65 are also known to co-regulate each other’s transcription. In summary, based on the bioinformatics analysis, NF-kB p65 and p53 could both potentially directly regulate transcription of SCO2 , TFAM , POLRMT , and CYB5A (Table 1 ; Supplementary Tables 1 and 2 ; Supplementary Fig. 8 ). Table 1 Bioinformatic analysis of putative-binding motifs for NF-κB and p53 Full size table To dismiss mitochondrial DNA (mtDNA) damage by EDCs as a possible mediator for mitochondrial insufficiency, mtDNA lesion measurements were performed using long-range quantitative PCR assay [51] , [52] . No significant lesions in mtDNA were observed in the presence of EDCs when compared with hydrogen peroxide-treated cells as a positive control (Supplementary Fig. 2g ). Cellular bioenergetics (ATP/ADP ratio) as reported by ATP levels were 25–50% lower in EDC-treated samples in both iFGEs and iHTNs (Fig. 5d ). The combination treatment elicited the strongest decrease in ATP levels ( p < 0.001; one-way ANOVA). Associating these findings to physiological endocrine disruption, levels of anorexigenic hormones in iFGEs, peptide YY (Fig. 5e ), and in iHTNs, secreted α-MSH (Fig. 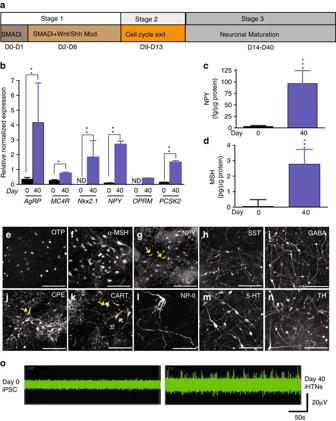Fig. 2 Functional neuropeptidergic hypothalamic neurons (iHTNs) can be derived from hiPSC.aiHTN differentiation protocol.bRT-qPCR of hypothalamic and arcuate nucleus-specific genes showing significantly increased expression of the genes at day 40 of differentiation compared with day 0 (*p< 0.05, **p< 0.01). ND not detectable; two-way ANOVA was employed to determine differences within day 0 and day 40 iHTNs.cMeasurement of hypothalamus-specific neuropeptide Y (NPY) measured from cell supernatants using ELISA (p< 0.001 determined using pairedt-test).dMeasurement of hypothalamus-specific α-melanocyte-stimulating hormone (α-MSH) measured from cell supernatants using ELISA (***p< 0.001 determined using pairedt-test).e–nImmunopositivity for hypothalamic progenitors and neuropeptidergic markers.oMEA readings of neurons from day 0 as well as day 40 from the same electrode over time showing increased neuronal firing in day 40 neurons. Images and data shown are representative of average results from the two iPSC lines differentiatedn= 5 times in independent experiments.Scale barsrepresent 50 µm.Error barsdenote s.e.m 5f ), were significantly decreased (20–55%) upon EDC treatment. Further, the levels of anorexigenic neuropeptide cocaine-regulated and amphetamine-regulated transcript (CART) were also negatively impacted upon EDC exposure of iHTNs (Supplementary Fig. 9a ). However, EDC exposure did not impart any significant changes in levels of orexigenic peptides, including AgRP or NPY (Supplementary Fig. 9 ). NF-κB inhibition rescues EDC-induced perturbations Considering that combination EDC exposures induced the most deleterious NF-κB pathway perturbations as well as mitochondrial dysfunction in the developing iPSC-endocrine cultures, we explored whether blocking NF-κB pathway with the cell permeable NF-κB peptide inhibitor (NF-κBi), SN50, can rescue these phenotypes. SN50 peptide inhibits nuclear induction of the NF-κB regulatory genes [53] . Upon co-treatment with EDCs and NF-κBi in the iFGEs and iHTNs, we found an overall decrease in phospho-p65, canonical (p50/p105), and non-canonical (p52/p100) pathway almost returning to the levels of the vehicle control (Fig. 6a, b ). NF-κBi did not appear to confer a specific inhibitory effect on p50 alone, but rather a more pan-inhibitory effect on activated p65, p50, and p52 levels in iFGEs (Fig. 6a ) and in iHTNs (Fig. 6b ) compared with combination treatment alone. NF-κBi treatment also decreased immune-positive pNF-κB cells induced by EDCs to levels of vehicle control (Fig. 6c ). Particularly, NF-κBi treatment also significantly improved the mitochondrial spare respiratory capacity of the combination EDC-treated cells (Fig. 6d ). The transcriptional regulation of mitochondrial respiratory genes, SCO2 , POLRMT , TFAM , and CYTB5 were also partially restored upon NF-κBi treatment compared with combination EDC treatment (Fig. 6e ). However, it is important to note that NF-κBi treatment did not rescue changes in ER stress proteins, IRE1, Ero1, and BiP (Supplementary Fig. 10a ), suggesting that ER stress may be upstream of the NF-κB pathway perturbations (Fig. 7 ). ATP levels also recovered significantly upon NF-κBi treatment in iFGEs and iHTNs (Fig. 6f ). Similarly, secretion of iHTN-derived anorexigenic hormone, α-MSH, also recovered upon NF-κBi treatment (Fig. 6g ). PYY levels in iFGEs were also restored upon NF-κBi treatment (Fig. 6h ). However, phosphorylation of p53 was not restored upon the NF-κB pathway inhibition suggesting that control of p53 phosphorylation may not be directly mediated via NF-κB in this paradigm (Supplementary Fig. 11a ). Fig. 6 Blocking NF-kB pathway rescues EDC-mediated metabolic stress and endocrine dysfunction. NF-kBi treatment decreases EDC-mediated increases in phosphorylated p65, p50, and p52 in a iFGEs and b iHTNs, * p < 0.05, ** p < 0.01, *** p < 0.001. Two different cell lines were loaded in 6 lanes with lanes 1, 2, and 3 belonging to 80iCTR (Vh1, Comb1, and NF-κBi1) and lanes 4, 5, and 6 from 201iCTR (Vh2, Comb2, and NF-κBi2). c Immunocytochemistry showing phosphorylated p65 staining in vehicle treatment ( Vh ), increased phospho-p65 with EDC combination treatment (Comb) that decreases with NF-κBi, * p < 0.05, ** p < 0.01, *** p < 0.001. d Seahorse assay showing improved mitochondrial respiration upon NF-κBi treatment compared with combination treatment in iHTNs, *** p < 0.001. e RT-qPCR expression levels of SCO2 , POLRMT , TFAM , and CYB5A showing decreased mitochondrial respiratory genes with combination treatment that are rescued by NF-κBi treatment, * p < 0.05, ** p < 0.01, *** p < 0.001. f Restoration of ATP levels upon NF-κBi treatment, ** p < 0.01, *** p < 0.001. g α-MSH secretion levels showed improvement upon NF-κBi treatment, *** p < 0.001. h Western blot showing rescue of PYY levels in iFGEs, * p < 0.05, ** p < 0.01. All statistical analysis performed using one-way ANOVA. Images and data shown are representative of average results from the two iPSC lines differentiated n = 3 times in independent experiments. Scale bars represent 50 µm. Error bars denote s.e.m Full size image Fig. 7 Proposed model of EDC-mediated dysregulation in developing endocrine tissues. Developing endocrine cells when exposed to EDCs such as PFOA, TBT, and BHT trigger endoplasmic reticulum (ER) stress by increasing IRE1 and downregulation of Ero1 and BiP, which are known to induce an unfolded protein response (UPR) in a cell. This results in perturbation of NF-κB (increased phosphorylation of p65) and p53 (decreased phosphorylation of p53 at Ser15) signaling in parallel. The subsequent metabolic stress is comprised of reduced transcription of both nuclear-encoded and mitochondrial-encoded respiratory genes, defective maximal respiration and mitochondrial spare respiratory, and a decrease in cellular bioenergetics/ATP levels. Intricate crosstalk between unhealthy mitochondria and ER may further lead to ER stress in a feedback loop and thereby exacerbate this mechanism. Overall, both accumulation of misfolded proteins as well as a decrease in ATP levels upon chronic exposure to low-dose of EDCs induces metabolic stress in an endocrine cell, thereby negatively impacting endocrine regulation because of abnormal production and secretion of gut and brain neuropeptides Full size image To the best of our knowledge, this is a previously undescribed finding linking the NF-κB pathway perturbation to ER stress and mitochondrial dysfunction upon stress challenge, especially in the context of endocrine disruption. There is a tremendous interest in better understanding the human exposome (a measure of insults from environmental exposures in an individual’s lifetime from before birth) and their consequences on human health. Americans are exposed to thousands of chemicals in our environment and more are introduced every day. EDCs like organotins, perfluorochemicals, and food additives that form a subset of this exposome are thought to be major contributors towards the obesity epidemic, viz. the “environmental obesogen” hypothesis [54] , [55] . Chronic exposure to obesogenic EDCs target hormonal signaling pathways in early endocrine system development and interfere with the cellular metabolic homeostasis. With the increasing prevalence of obesity in child-bearing individuals, the developmental programming of the fetus has been shown to be more susceptible to alterations in endocrine system and metabolic development, and predisposing offspring to metabolic disorders [56] . Many EDCs continue to pose health hazards, as in 2016, Alabama discovered the presence of significant levels of PFOA in drinking water sourced from the Tennessee river despite efforts on phasing out its as per Environmental Protection Agency’s (EPA’s) request [57] . Efforts are also ongoing to remove BHT as an antioxidant additive in breakfast cereals. There is enormous public interest in examining the health risk posed by these “everywhere chemicals”. Given that a daily exposure to EDCs may lead to long-term endocrine disruption and metabolic dysfunction during development, the impact of EDCs in relevant human endocrine cell platforms needs to be determined. Accessing human fetal tissue at different developmental stages upon exposure to EDCs is implausible. Therefore, in this study, we addressed this gap by using human pluripotent stem cell-derived endocrine tissue, i.e., brain neuroendocrine cells (iHTNs) and gut endocrine cells (iFGEs). Briefly, here we describe reliable methods to create these relevant endocrine-active gut and brain cultures from iPSCs, and demonstrate the adverse impacts of three different EDCs pervasive in food and household items. The chronic exposure of three different EDCs (PFOA, TBT, and BHT) at physiologically relevant low-doses, to human iPSC-endocrine cells is detrimental to early endocrine cell function without negatively impacting endocrine cell differentiation. We discovered that ER stress is a major early driver in the EDC-mediated perturbations in both iFGEs and iHTNs. ER stress sensor and activator of UPR, IRE1, was increased, whereas molecular chaperone and folding proteins, BiP/GRP78 and Ero1, were markedly attenuated upon EDC treatment. As many secreted proteins and peptide hormones undergo protein folding process mediated by BiP and Ero1 to reach their native conformation and fold properly, the decrease in these proteins suggest accumulation of misfolded proteins as a compensatory mechanism when ER stress is activated [58] . Downstream of EDC-induced ER stress, we assessed whether EDC treatment altered NF-κB signaling. In general, the NF-κB pathway has been well-studied in inflammatory processes, cancer biology, and tumor progression [59] , but little is known with regard to its role in endocrine regulation, developmental programming, and cell metabolism. RelA/p65 is part of the classical canonical NF-κB pathway known to be stimulated by cytokines such as tumor necrosis factor-α (TNF-α) or other infectious agents, and depends on the degradation of IκB via its ubiquitination that leads to p65:p50 dimers thereby activating this pathway [60] , [61] . Here, we demonstrated that EDC exposure significantly increased phosphorylation of p65 in iHTN and iFGE endocrine tissues, suggesting a possible common mechanism of endocrine disruption across this class of chemicals. Consequently, EDC exposures increased processing of p105 to p50 as well as p100 to p52, suggesting activation of both canonical and non-canonical NF-κB signaling pathways. p65/RelA is involved in transactivation of both p105 [62] and p100 [60] promoters, thus serving as a common activator of the canonical and non-canonical pathways. Although confirmatory studies in animal models are required, this finding of EDC-induced perturbation of NF-κB signaling in developing brain and gut tissues could implicate long-term adverse effects on neuroendocrine and food-intake circuitries. To the best of our knowledge, this is the first report demonstrating that EDCs can uniformly perturb the NF-κB pathway. Evidence from the literature suggests that ER stress with inputs from IRE1 can directly activate NF-κB p65 (RelA) by integrating IRE, PERK, and IKK functions [41] . ER stress was likely upstream pathway of NF-κB activation as it was unaffected by blocking NF-κB signaling. The EDC-mediated ER stress molecules involved in an UPR could also have a role in the decrease in precisely regulated secretion of α-MSH in iHTNs and PYY in iFGEs. Furthermore, phosphorylated p53 (Ser15) decreased upon EDC treatment without changes in the total p53 protein levels, and this molecular change could not be rescued by the NF-κB pathway inhibition (Supplementary Fig. 9a ). This suggests that upon EDC exposure p53 possibly functions either upstream or in concert with NF-κB in the developmental stem cell-derived endocrine culture systems (Fig. 7 ).This is also supported by evidence that loss of p53 is involved in the phosphorylation of NF-kB p65 [61] . An interesting aspect of this study revealed unfavorable alterations in cellular metabolic health and mitochondrial respiratory capacity engendered by EDCs. Decrease in mitochondrial function is involved in long-term metabolic dysfunction in obesity and type 2 diabetes, and NF-κB signaling is associated with mitochondrial function via crosstalk through p65, p100, and p105 proteins [50] . There were differing impacts of each EDC on the mitochondrial respiratory capacity in both endocrine cell cultures. In the iFGEs, only BHT and combination treatments produced a significant decrease in the mitochondrial spare respiratory capacity upon a stress test with carbonyl cyanide- p -trifluoromethoxyphenylhydrazone (FCCP, an uncoupling agent that disrupts ATP synthesis), whereas in the iHTNs, TBT, BHT, and combination treatments engendered a similar effect. Although the entire set of EDC treatments perturbed NF-κB signaling, perhaps longer exposures of PFOA are required to impart sustained mitochondrial effects. These mitochondrial abnormalities were associated with NF-κB signaling impairments, as EDC exposures also downregulated transcription of known NF-κB responsive genes involved in mitochondrial function, namely: SCO2 (subunit of cytochrome c oxidase), POLRMT (Mitochondrial RNA polymerase), TFAM (Transcription factor A, mitochondrial), all of which are nuclear-encoded, and CYB5A (Cytochrome B5) that is mitochondrially encoded. NF-κB affects oxidative phosphorylation, glycolysis, and ATP production via nuclear and mitochondrial gene expression ( TFAM and POLRMT ) through a crosstalk between NF-κB RelA (p65) and other transcription factors [50] , [63] . Furthermore, RelA likely directly translocates to mitochondria and represses mitochondrial gene expression thereby downregulating oxidative phosphorylation [50] . Knocking down RelA increased binding of POLRMT to the D-loop of mitochondrial genome, increased CYB5A mRNA levels and increased ATP production and recruitment of p65 to mitochondrial genome and its C-terminal transactivation domain repressing POLRMT binding to mtDNA [64] . CYB5A (CytB5), a mitochondrially encoded gene has also been previously shown to be regulated by NF-κB [65] . The bioinformatics analysis presented here identified putative DNA binding sites for p65 as well as p53 near the transcription start site of these mitochondrial respiratory genes, suggesting that both p65 and p53 also regulate their transcription. Thus, the perturbation of post-translational modifications (phosphorylation) in p65 and p53 also may lead to repression of respiratory gene expression. There is also a direct link between ER stress, mitochondrial dysfunction and metabolic stress via transactivation of mitochondrial genes and NF-κB-mediated repression of mitochondrial gene expression [58] . Other evidence points to p65-mediated negative regulation of gene transcription via interaction with histone deacetylase [66] . To the best of our knowledge, with respect to p53, there is no direct evidence describing its direct regulation of mitochondrial DNA-encoded gene expression. However, p53 is inhibited in response to ER stress [67] . In this cellular model, EDC exposure disrupted p65 and p53 signaling to decrease expression of mitochondrial respiratory genes like CYB5A and POLRMT , and attenuated cellular respiratory capacity. Employing a co-treatment with NF-κB cell permeable peptide inhibitor, SN50, significantly decreased the EDC-induced increases in phosphorylated p65 and increased processing to p50 and p52. In line with this, suppressing p65 phosphorylation blocked abnormalities in mitochondrial respiratory gene expression and function, thus linking the impairment of mitochondrial function to the NF-κB pathway perturbation. In general, this mechanistic link has been under-explored, especially in the context of endocrine disruption. Thus, we posit that the increase in NF-kB p65 phosphorylation and a decrease in p53 phosphorylation upon EDC treatment, together regulates transcription of genes regulating cellular bioenergetics, and negatively affects the metabolic function in endocrine cells. It is, however, important to keep in mind that the mitochondrial dysfunction brought about by changes in NF-κB p65 and p53 pathways was accompanied by decreases in maximal mitochondrial respiration and ATP levels. This, we believe, could also have a direct effect on the packaging and secretion of hormones by an endocrine cell. As hormone production and secretion is an ATP-dependent process, compromised bioenergetics impacts this process. EDCs caused decreases in levels of secreted anorexigenic neuropeptide, α-MSH, as well CART neuropeptide. However, EDCs did not produce any differences in AgRP or secreted NPY neuropeptide levels. This suggest that EDC exposure preferentially negatively targets pathways controlling anorexigenic responses, thereby possibly tilting the overall cellular milieu to be orexigenic. Similarly, in the hiPSC-derived gut-epithelium, the anorexigenic peptide YY levels declined upon EDC exposure. These changes could be attributed to either ER stress-mediated mitochondrial dysfunction and decreases in ATP production as described above and/or concurrent activation of the UPR pathways. Intricate crosstalk between unhealthy mitochondria and a stressed ER-mediated UPR may exacerbate this process in endocrine tissues, further compounding the mitochondrial insufficiency and metabolic stress, and negatively impacting production and secretion of gut–brain hormonal peptides during critical periods of early human development (Fig. 7 ). In summary, we apply the human pluripotent stem cell platform towards predictive endocrine toxicology of pervasive EDCs. The metabolic stress induced by EDCs tested here, PFOA, TBT, and BHT, was comprised of ER stress activation, abnormal p65 and p53 signaling, reduced transcription of both nuclear-encoded and mitochondrial-encoded respiratory genes, defective maximal respiration and mitochondrial spare respiratory, decrease in cellular bioenergetics/ATP levels, and subsequent endocrine dysregulation as demonstrated by aberrant production and secretion of peptide hormones. Although it remains to be demonstrated how long-term ER stress, perturbation of NF-κB p65 and p53 signaling, and mitochondrial dysfunction in developing endocrine cells may contribute to metabolic diseases like obesity and type 2 diabetes, the platform described here has enormous potential for screening the developmental impact of human exposure to harmful endocrine disrupting chemicals in the environment. Ethics statement and reprogramming to iPSCs Human PBMCs were obtained from whole-blood draws of healthy volunteers at Cedars-Sinai under the auspices of the Cedars-Sinai Medical Center Institutional Review Board (IRB) approved protocol Pro00028662. The reprogramming and characterization of iPSC cell lines and differentiation protocols in the present study were carried out in accordance with the guidelines approved by Stem Cell Research Oversight committee (SCRO) and IRB, under the auspices of IRB-SCRO Protocols Pro00032834 (iPSC Core Repository and Stem Cell Program) and Pro00036896 (Sareen Stem Cell Program). Briefly, for reprogramming, PBMCs were maintained in RPMI 1640 (Life Technologies) supplemented with 15% FBS and 2mM l -glutamine cultured at 37 °C and 5% CO 2 . Reprogramming was performed using virus-free episomal plasmids (Addgene) with nucleofector Kit C (VACA01004, Lonza) to express OCT4, SOX2 , KLF4 , L-MYC , LIN28 , SV40LT and p53 shRNA (pEP4 E02S ET2K, pCXLE-hOCT3/4-shp53-F, pCXLE-hUL, and pCXLE-hSK). Appropriate informed consents were obtained from all the donors. To protect donor privacy and confidentiality, all samples were coded and de-identified in this study. Human iPSC culture and quality control Human iPSCs that were maintained under feeder-free culture conditions in growth factor reduced Matrigel and defined lab-made Essential 8 (E8) media. The iPSCs were passaged every 5–7 days using the StemPro EZ Passaging Tool (Life Technologies) or Versene solution (Life Technologies). Every cell line in the iPSC core cultured is tested monthly for mycoplasma using the MycoAlert™ PLUS Mycoplasma Detection Kit (Lonza; LT07-710). Our annual rate of mycoplasma contamination is <0.2% and only mycoplasma-free cell lines were used in this study for analysis. The iPSC lines once reprogrammed were authenticated using cell line identity assay by short tandem repeat (STR) profiling, and compared with parental tissue source (PBMCs). For STR profiling, the iPSC lines were authenticated by the Cedars-Sinai iPSC Core by contracting with IDEXX Laboratories, Inc. and use of their CellCheck 9 service. This test allows provides a human 9 STR marker profile and for interspecies contamination check for human, mouse, rat, African green monkey, and Chinese hamster cells. The identity of all cell lines validated is matched to tissue source annually and at the time of generation of the distribution cell bank. Certificate of Analysis of all iPSC lines used in this manuscript are available upon request from the Cedars-Sinai iPSC Core. Foregut epithelium differentiation (iFGE) For differentiation, iPSCs were accutase-treated and plated into a 6-well Matrigel-coated dish at a density of 1x10 6 per well in E8 medium with ROCK-inhibitor Y27632 (10 μM; Stemgent). On the next day, iPSCs were differentiated into definitive endoderm by exposing them to Activin A (100 ng/ml; R&D) and Wnt3A (25 ng/mL only on the first day; Peprotech) in RPMI 1640 (Gibco) for 3 days. During these 3 days, the cells were exposed to increasing concentrations of 0, 0.2, and 2% defined FBS (dFBS, Hyclone). After definitive endoderm induction, the cells were directed to form foregut spheroids by culturing them for the next 3 days in Advanced DMEM/F12 medium (Gibco) containing 2% dFBS, 2 μM CHIR99021 (2 μM; Cayman), FGF4 (500 ng/mL; Peprotech), LDN193189 (2 μM; Cayman), and retinoic acid (2 μM; Cayman). This resulted in semi floating spheroids, which were then selectively picked and transferred on to Matrigel-coated experimental plates for further maturation and experimentation. For maturing the picked foregut spheroids, they were cultured in a medium containing Advanced DMEM/F12 with N2 (Invitrogen), B27 (Invitrogen), GlutaMax, Penicillin/streptomycin/Antimycotic, and EGF (100 ng/ml; Peprotech). Media was replaced every 2–3 days as necessary and the spheroids are allowed to develop into an epithelial monolayer until day 20. Hypothalamic neuron differentiation (iHTN) For differentiation into iHTNs, iPSCs were accutase-treated and plated as single cells in 6-well Matrigel-coated plates at a density of approx. Overall, 1x10 6 cells per well in E8 medium with ROCK-inhibitor Y27632 (10 μM; Stemgent). The next day iHTN differentiation was initiated by neuroectoderm differentiation by dual SMAD inhibition using LDN193189 (1 μM, Cayman) and SB431542 (10 μM, Cayman) and this treatment is carried on for 48 h. This was followed by Sonic hedgehog activation by Smoothened agonist SAG (1 μM, Tocris) and purmorphamine (PMN, 1 μM, Tocris) and Wnt signaling inhibition using IWR-endo (10 μM, Cayman) from day 3 to 8 to direct the cells towards ventral diencephalon with regular media change every 2 days. From day 9 to 13, the cells are slowly made to exit cell cycle using DAPT (10 μM, Cayman) in the presence of ventralizing agent retinoic acid (0.1 μM, Cayman). On day 14, the cells were treated with Accutase and re-plated onto laminin-coated plates in the presence of maturation medium containing brain-derived neurotrophic factor BDNF (10 ng/mL, Miltenyi) and maintained until day 40. EDC treatments We employed three different EDCs, Perfluoro-octanoic acid (PFOA) (2.5 μM, Sigma-Aldrich), Tributyltin (TBT) (10 nM, Sigma-Aldrich) and butylated hydroxytoluene (BHT) (10 nM, Cayman) individually and in combination. We hence had six treatment groups namely Vehicle control (Vh), PFOA, TBT, BHT, and combination treatment. iFGE treatment of EDCs was carried out by performing the differentiation as mentioned above and adding EDC treatments during the final 12 days of differentiation, i.e., day 8 to 20. Similarly, iHTNs were differentiated as per the protocol detailed above and the final 12 days of differentiation, i.e., day 28 to 40 EDC treatments were performed. For the rescue experiments using NF-κBi (SN50), the cells were first exposed to NF-κBi 24 h before EDC treatment. Subsequently, the cells were treated with the combination treatment along with NF-κBi where NF-κBi treatment was combined with combination EDC-treated conditions. Immunofluorescence Cells that were subject to immunofluorescence were first fixed using 4% paraformaldehyde (PFA) for 20 min and subsequently washed with PBS. After blocking the cells with 5% donkey serum (Millipore) with 0.2% triton X-100 (Bio-rad) in PBS for a minimum of 2 h, the cells were then treated with an appropriate concentration of relevant primary antibody combinations (1:250) overnight at 4 °C. After thorough washing using PBS with 0.1% Tween-20, the cells are then treated with appropriate species-specific Alexa Fluor-conjugated secondary antibody combinations for 45 min (1:500). Hoechst stains were used to mark the nuclei and the cells were then visualized using appropriate fluorescent filters using ImageXpress Micro XLS (Molecular devices). 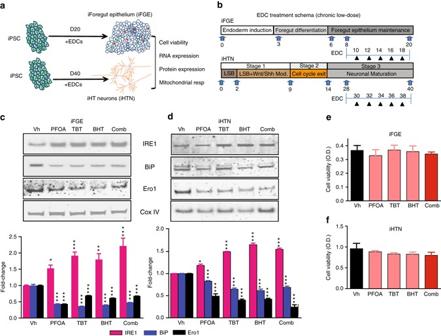Fig. 3 Chronic low-dose EDC treatment induces ER stress in iFGEs and iHTNs without affecting cell viability.aA schematic representation of EDC treatments and analysis performed on iFGEs and iHTNs.bA schematic showing the kinetics of EDC treatments performed on iFGEs and iHTNs.c,dRepresentative immunoblots showing levels of bona fide ER-stress pathway proteins, IRE1, BiP, and Ero1, inciFGE anddiHTNs. Quantified histograms using ImageJ-based densitometry of bands for each of the respective protein immunoblots normalized to Cox IV as loading control are shown below and represented as fold-change compared with vehicle-treated control. IRE1 protein increases, whereas BiP and Ero1 levels decrease in response to EDC exposure, *p< 0.05, **p< 0.01, ***p< 0.001.e,fMTT assay shows no significant differences in cell viability upon EDC exposure in botheiFGEs andfiHTNs. All statistical analyses were performed using one-way ANOVA. Data shown are representative of average results from the two iPSC lines differentiatedn= 3 times in independent experiments.Error barsdenote s.e.m Antibodies and dilutions employed can be found in Supplementary Table 3 . Immunoblots Cell pellets were collected and lysed (mammalian PER, Thermo scientific + 1x protease inhibitor cocktail, Thermo Scientific), and samples were prepared after protein quantification. We loaded about 15 µg protein per lane of a polyacrylamide gel (NuPAGE™ Novex™ 4–12% Bis-Tris Protein Gels). Once the gels were resolved, they were transferred onto nitrocellulose membrane and subsequently blocked in 5% milk solution for a minimum of 2 h. This was followed by a one-step i-Bind process which treated the membrane with primary antibody, washing and secondary antibody steps (Life technologies). We employed LiCor® IRDye secondary antibodies (680 and 800 wavelength infrared dyes) and detection of bands was carried out in a LiCor ODyssey CLx imager (LiCor). Antibodies and dilutions employed can be found in Supplementary Table 3 . Full blots are provided in Supplementary Figs. 4 and 5 . Quantitative PCR Total RNA was isolated using the RNeasy Mini Kit (Qiagen) and RNA (2 μg) was first DNase treated and reverse transcribed to cDNA with oligo(dT) using the Promega Reverse Transcriptase System (Promega). Reactions were performed in three replicates using SYBR Green master mix (Applied Biosystems) using primer sequences specific to each gene. Each PCR cycle consisted of 95 °C for 10 min, 95 °C 30 ss → 58 °C for 60 s, for 50 cycles, and 72 °C for 5 min. Genes of interest were normalized to either RPL13A or 16srRNA for mitochondrial genes. 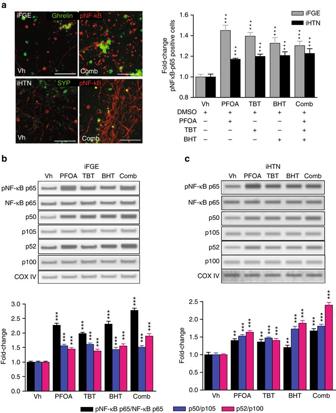Fig. 4 EDC treatment causes disturbances in NF-κB p65 canonical and non-canonical pathways.aTop panel: representative immunocytochemistry (ICC) showing increases in phosphorylated p65 (red) in iFGEs co-stained with ghrelin (green).Bottom panel: representative ICC showing increases in phosphorylated p65 (red) in iHTNs co-stained with synaptophysin (green) (***p< 0.001). Immunopositive cells were scored and quantified in histograms for both iFGEs and iHTNs, which is represented by fold-change in phosphorylated NF-κB p65 immunopositive cells in each of the EDC treatments compared with the vehicle control-treated iFGEs (***p< 0.001) and iHTNs (***p< 0.001). Representative immunoblots for protein levels in whole-cell lysate showing increases in phosphorylated p65, total p50, and total p52 levels inbiFGE, ***p< 0.001 andciHTNs ***p< 0.001. Quantified histograms using ImageJ-based densitometry of bands for each of the respective immunoblots are shown below and represented as fold-change compared with vehicle-treated control. Ratio of phosphorylated NF-κB p65 over total p65, p50/105 (canonical), and p52/p100 (non-canonical) were calculated. All statistical analyses were performed using one-way ANOVA. Images and data shown here are representative of average results from the two iPSC lines differentiatedn= 3 times in independent experiments.Scale barsrepresent 50 µm.Error barsdenote s.e.m Primer sequences can be found in Supplementary Table 4 . MTT assay Cell viability was assessed by MTT assay. Cells were plated in 96-well plates at a density of 10,000 cells in 100 μL medium per well. On the day of assay, fresh media was added (100 μL) and 10 μL MTT solution was added to the culture medium (12 mM stock MTT solution) and incubated at 37 °C for 4 h. The reaction was stopped by the addition of 50 μL DMSO to each well. Wells lacking any cells were included as a negative control to subtract background. The absorbance value was read at 540 nm using an automatic multi-well spectrophotometer (Perkin Elmer). 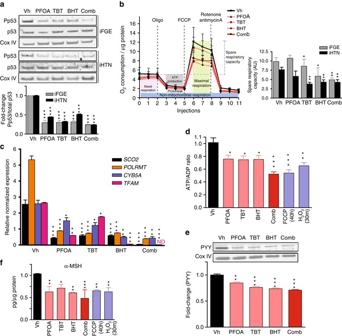Fig. 5 EDCs induce metabolic stress and disrupt endocrine regulation.aImmunoblots showing decreases in phosphorylated p53 (Ser15) in both iFGEs and iHTNs (***p< 0.001) upon EDC exposure.bSeahorse mitochondrial respirometry measurements with histograms representing changes in spare respiratory capacity in iFGEs and iHTNs, *p< 0.05; **p< 0.01.cRelative normalized expression of nuclear (SCO2, POLRMT, TFAM) and mitochondrial-encoded (CYB5A) genes involved in mitochondrial respiration in iHTNs as measured by RT-qPCR.dMeasurement of ATP levels (ATP/ADP ratio) showing decreases with EDC treatments.eImmunoblots showing decreases in PYY levels in EDCs-treated iFGEs.fELISA of α-MSH showing decreases in secretion with EDC treatment of iHTNs. *p< 0.05, **p< 0.01, ***p< 0.001,n= 3. ND not detectable. All statistical analysis was performed using one-way ANOVA. Data shown here are representative of average results from the two iPSC lines differentiatedn= 3 times in independent experiments.Error barsdenote s.e.m Metabolic phenotyping and seahorse respirometry assay The Seahorse XF e 24 Extracellular Flux Analyzer (Seahorse Biosciences) was used to perform mitochondrial stress tests and obtain real-time measurements of oxygen consumption rate (OCR) in cells. iFGEs and iHTNs treated with or without EDCs were seeded in a 24-well Seahorse culture plate at a density of 10,000–15,000 cells per well. For analysis of OCR, cells were reconstituted in Seahorse-base medium and were allowed to settle for 1 h at 37 °C in non-CO 2 incubator before measurements. Chemical reagents (Sigma) were used at final concentrations as follows: 1 μM oligomycin—an ATP synthase inhibitor, 1 μM (FCCP) carbonyl cyanide 4-(trifluoromethoxy)phenylhydrazone—an uncoupling agent, and a mixture of 0.5 μM antimycin A—a cytochrome C reductase inhibitor and 0.5 μM rotenone—a complex I inhibitor. Results were normalized to protein concentration determined by BCA assay (Thermo Scientific). Mitochondrial DNA integrity assay Quantitative polymerase chain reaction (QPCR) was employed to determine mitochondrial DNA damage by measuring DNA lesions in the mitochondrial DNA. Lesions tend to slow down the progression of DNA polymerase [68] and therefore the greater the lesions, the lesser the amplification. Here the long-range PCR assay was utilized, which involves the isolation of high molecular weight genomic DNA (Qiagen). Using Pico green dye (Thermo Fisher) and Lambda/Hind III DNA (Thermo Fisher) the DNA yield was quantified. PCR was performed using the Elongase Enzyme Mix (Thermo Fisher). qPCR was performed based on the protocol by Santos et al [52] . Pico green was used to quantify the amplification efficiency of the PCR products. To measure mitochondrial lesions, we employed a small and a large mitochondrial primer to amplify and short and a long fragment of the mitochondrial DNA, respectively. The amplification of the small mitochondrial fragment was used as a measure of total amount of mitochondrial DNA, whereas the amplification efficiency of the large mitochondrial fragment was used as a measure of lesions. In other words, the less the amplification, the greater the lesions [52] . Identification of putative-binding motifs for p65 and p53 To identify possible binding sites for the p65 and TP53 transcription factors, we searched for sequences upstream of our genes of interest, which matched the binding motifs of our transcription factors. We accomplished this by following methods outlined in the Bioconductor workflow “Finding Candidate Binding Sites for Known Transcription Factors via Sequence Matching”. This workflow describes a method for identifying the nucleotide-binding motif for transcription factors using the UCSC hg19 annotation of the human genome. Because the protein binding motifs bind more consistently with specific nucleotides at specific positions, these binding motifs are saved as a set of positional weight matrices. Possible binding sites can be determined using the match PWM function in the Biostrings package. The number of hits detected depends on the length of the upstream sequence provided and the specificity cutoff supplied by the user. We searched for possible binding sites in the 2000 bp upstream of our transcription start sites using specificities set at 60, 70, 80, and 85%. We performed this check against our genes of interest, as well as genes known to be promoted by our transcription factors, as well as fifty random genes, which we assume have no unique association to our transcription factors. ATP/ADP ratio assay ATP/ADP ratio assay was carried out using Enzylight™ ADP/ATP Ratio Assay kit (BioAssay Systems; Cat # ELDT-100) as per manufacturer’s instructions. The principle of this bioluminescence assay is based on a 2-step protocol where the first step involves the release of ATP and ADP. ATP readily reacts with luciferase in the presence of substrate d -luciferin, which produces light and is a direct measure of the intracellular ATP concentration. The second step involves a kit contained enzyme-mediated conversion of ADP to ATP. This newly formed ATP again reacts with d -luciferin and produces a new set of luminescent values. The two values were then utilized to calculate ATP/ADP ratio using the following formula. ATP/ ADP ratio= RLU A/( RLU C -  RLU B),
 where RLU A is the relative luminescence unit of ATP, RLU B is the measurement after 10 min of RLU A measurement to provide a background reading for ADP measurement, and RLU C is the luminescence of ADP. α-MSH ELISA We employed the Cloud-Clone Corp enzyme-linked immunosorbent assay (ELISA) kit (Cat # CEA239Hu) to measure secreted levels of α-MSH from our cell supernatants. This competitive inhibition enzyme immunoassay technique uses a monoclonal α-MSH antibody pre-coated microplate, which launches a competitive inhibition reaction between biotin-labeled α-MSH and the unlabeled α-MSH from standard and samples. An avidin-conjugated Horseradish peroxidase helps identify the unbound sites within each sample and the substrate-mediated color development is inversely proportional to the concentration of α-MSH in the sample. A log–log graph was used to quantify the amount of α-MSH present in each sample. NPY ELISA We employed the EMD Millipore Human Neuropeptide Y ELISA kit (Cat # EZHNPY-25K) to measure secreted NPY levels. This is a sandwich ELISA that captures NPY in the sample by antihuman NPY IgG and immobilizes the resulting complex to wells of a microtiter plate coated with pre-titered amount of anchor antibodies. The captured NPY then binds to a second biotinylated antibody to NPY followed by conjugation of horseradish peroxidase to the immobilized biotinylated antibodies. NPY is quantified by monitoring horseradish peroxidase activities in the presence of the substrate 3,3′,5,5′-tetra-methylbenzidine. 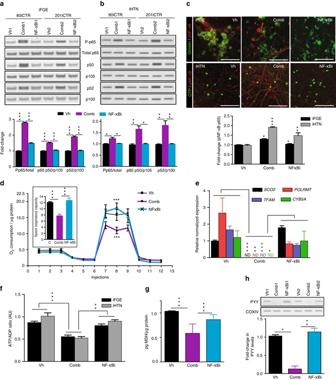Fig. 6 Blocking NF-kB pathway rescues EDC-mediated metabolic stress and endocrine dysfunction. NF-kBi treatment decreases EDC-mediated increases in phosphorylated p65, p50, and p52 inaiFGEs andbiHTNs, *p< 0.05, **p< 0.01, ***p< 0.001. Two different cell lines were loaded in 6 lanes with lanes 1, 2, and 3 belonging to 80iCTR (Vh1, Comb1, and NF-κBi1) and lanes 4, 5, and 6 from 201iCTR (Vh2, Comb2, and NF-κBi2).cImmunocytochemistry showing phosphorylated p65 staining in vehicle treatment (Vh), increased phospho-p65 with EDC combination treatment (Comb) that decreases with NF-κBi, *p< 0.05, **p< 0.01, ***p< 0.001.dSeahorse assay showing improved mitochondrial respiration upon NF-κBi treatment compared with combination treatment in iHTNs, ***p< 0.001.eRT-qPCR expression levels ofSCO2,POLRMT,TFAM, andCYB5Ashowing decreased mitochondrial respiratory genes with combination treatment that are rescued by NF-κBi treatment, *p< 0.05, **p< 0.01, ***p< 0.001.fRestoration of ATP levels upon NF-κBi treatment, **p< 0.01, ***p< 0.001.gα-MSH secretion levels showed improvement upon NF-κBi treatment, ***p< 0.001.hWestern blot showing rescue of PYY levels in iFGEs, *p< 0.05, **p< 0.01. All statistical analysis performed using one-way ANOVA. Images and data shown are representative of average results from the two iPSC lines differentiatedn= 3 times in independent experiments.Scale barsrepresent 50 µm.Error barsdenote s.e.m 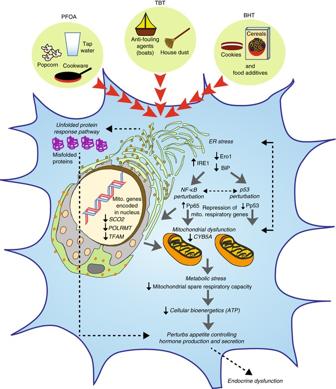Fig. 7 Proposed model of EDC-mediated dysregulation in developing endocrine tissues. Developing endocrine cells when exposed to EDCs such as PFOA, TBT, and BHT trigger endoplasmic reticulum (ER) stress by increasing IRE1 and downregulation of Ero1 and BiP, which are known to induce an unfolded protein response (UPR) in a cell. This results in perturbation of NF-κB (increased phosphorylation of p65) and p53 (decreased phosphorylation of p53 at Ser15) signaling in parallel. The subsequent metabolic stress is comprised of reduced transcription of both nuclear-encoded and mitochondrial-encoded respiratory genes, defective maximal respiration and mitochondrial spare respiratory, and a decrease in cellular bioenergetics/ATP levels. Intricate crosstalk between unhealthy mitochondria and ER may further lead to ER stress in a feedback loop and thereby exacerbate this mechanism. Overall, both accumulation of misfolded proteins as well as a decrease in ATP levels upon chronic exposure to low-dose of EDCs induces metabolic stress in an endocrine cell, thereby negatively impacting endocrine regulation because of abnormal production and secretion of gut and brain neuropeptides The enzyme activity is measured spectrophotometrically by the increased absorbency at 450 nm. The increase in absorbency is directly proportional to the amount of captured NPY. Statistical analysis In this study, we report perturbations induced by endocrine disrupting chemicals on developing endocrine tissues. Experiments were performed using two independent donor-derived iPSC lines on gut endocrine cultures (iFGEs) and HTNs. Multiple differentiations and treatments performed in independent experiments and are stated in each figure legend. All data are represented as mean ± s.e.m. p values < 0.05 were considered significant—* p < 0.05, ** p < 0.01, *** p < 0.001 and **** p < 0.0001. All statistical analyses were performed on GraphPad Prism using student’s unpaired t -test (with or without Welch’s correction) or one-way Analysis of variance (ANOVA) and Bonferroni post-test for multiple comparisons. Code availability The Bioconductor workflow Identification of Putative-Binding Motifs and Transcription Start Sites for p65 and p53 can be found at: https://www.bioconductor.org/help/workflows/generegulation/ . The R script used in this study can be found on Github at: https://github.com/andrewrgross/Activation-site-identification Data availability The data that support the findings of this study are available from the corresponding author upon reasonable request.